Small palladium islands embedded in palladium–tungsten bimetallic nanoparticles form catalytic hotspots for oxygen reduction The sluggish kinetics of the oxygen reduction reaction at the cathode side of proton exchange membrane fuel cells is one major technical challenge for realizing sustainable solutions for the transportation sector. Finding efficient yet cheap electrocatalysts to speed up this reaction therefore motivates researchers all over the world. Here we demonstrate an efficient synthesis of palladium–tungsten bimetallic nanoparticles supported on ordered mesoporous carbon. Despite a very low percentage of noble metal (palladium:tungsten=1:8), the hybrid catalyst material exhibits a performance equal to commercial 60% platinum/Vulcan for the oxygen reduction process. The high catalytic efficiency is explained by the formation of small palladium islands embedded at the surface of the palladium–tungsten bimetallic nanoparticles, generating catalytic hotspots. The palladium islands are ~1 nm in diameter, and contain 10–20 palladium atoms that are segregated at the surface. Our results may provide insight into the formation, stabilization and performance of bimetallic nanoparticles for catalytic reactions. The world’s rapidly growing demand for energy and the requirement of sustainable energy production calls for an urgent change in today’s fossil fuel-based energy system [1] , [2] . Vast efforts are invested by research groups worldwide to develop and study novel advanced energy conversion and storage systems with high efficiency, low cost and environmental compatibility. Fuel cell systems, such as proton exchange membrane fuel cells, using oxygen as oxidant, represent a promising alternative for low carbon emission energy production [3] , [4] , [5] . Historically, platinum and its alloys have frequently been used as anodic and cathodic catalysts in fuel cells owing to their high activity for fuel oxidation and oxygen reduction reactions (ORRs). However, the high cost of platinum, owing to its low abundance and to limited mining capabilities [6] , in combination with a high sensitivity of platinum towards reaction intermediates or fuel impurities has accelerated the search for cheaper and more efficient catalyst materials [7] . A recent major achievement is the reduced need of expensive noble metals by the use of nanoparticles [8] , [9] , [10] , [11] , [12] , and by attaching and stabilizing these on conducting supports with large surface area, such as carbon fibres [13] , carbon nanotubes [14] , graphene [15] and mesoporous carbon [16] , [17] . Some studies have even shown the possibility to completely avoid the use of noble metals by the use of nitrogen-doped carbon nanostructures [18] , [19] . Still, however, the motivation is very high to develop new high-performance systems with low cost and good stability. One of the most recent topics, which has attracted significant interest, is the development of bimetallic nanoparticles composed of mixtures of noble metals and inexpensive metals such as tungsten (W), cobalt or nickel [20] , [21] . Some key studies have demonstrated that bimetallic core-shell nanoparticles with the noble metal as the shell can demonstrate excellent catalytic activity, which sometimes even outperform commercial single-metal catalysts [22] , [23] , [24] , [25] , [26] , [27] . However, in certain cases, the synthesis of core-shell particles is difficult to achieve. Furthermore, core-shell particles set a lower limit on the ratio of noble metals in the bimetallic nanoparticle, since the amount of noble metal must be sufficient to form a continuous shell. Here we report the design of bimetallic nanoparticles in which a high electrocatalytic activity for ORRs does not rely on the formation of core-shell nanoparticles but rather on the formation of few-atomic palladium (Pd) islands embedded in Pd–W nanoparticles. The bimetallic nanoparticles are supported on ordered mesoporous carbon (OMCs) that assures a high surface area, good conductivity and good diffusion of oxygen in the catalyst. The ordered pores with a narrow size distribution of the OMCs also efficiently limits the size of the catalyst nanoparticles, which gives the highest possible utilization of the noble metals [28] . The synthesis is performed in a regular kitchen microwave oven in less than a minute. The formation of the Pd islands are supported by experimental and theoretical data, and confirmed by extended X-ray absorption fine structure spectroscopy (EXAFS), which based on a coordination number analysis demonstrate that the embedded Pd islands contain 10–20 atoms on average. We further show that Pd islands embedded in the W-matrix are metallic, and despite their small size (~1 nm) they are remarkably stable, explained by the reducing environment of the W-matrix. By implementing our Pd–W/OMCs as cathode catalysts in a fuel cell, we observe a performance similar to that obtained with a commercial catalyst (60% Pt/Vulcan) at a noble metal cost being 40 times lower. The high catalytic activity is rationalized by positive synergy effects from the surrounding W atoms in combination with the reducing environment of W, which efficiently keeps the Pd atoms metallic and catalytically active. The experimental findings are well supported by density functional theory (DFT) calculations showing that some configurations of the Pd islands may have comparable catalytic efficiency as pure Pt (111) surfaces. Our results provide insight into the formation, stabilization and performance of a novel bimetallic type of nanoparticles for catalytic reactions, where a complete core-shell configuration is not crucial for high-performance, cost-efficient electrocatalysts. This may lead to other designs of bimetallic nanoparticles in the future. Physical properties of Pd–W/OMC catalyst The preparation of the catalyst is performed by a microwave-assisted synthesis, which avoids the problems of a hydrophobic OMCs support and hydrophilic catalyst salts [29] , and is pursued without any use of carbon support functionalization or polymer coating of nanoparticles as previously utilized to overcome this problem [30] . The synthesis is schematically described in Fig. 1a . Pd(OAC) 2 is mixed with W(CO) 6 in toluene. Thereafter, OMCs is added and the mixture is ground in a mortar. The mixture is placed in a vial, purged with argon and then treated in a regular microwave oven for 1 min. During the synthesis, the Pd and W precursors penetrate into the porous OMCs during solvent evaporation. The colour of the sample radiates with yellow–red colour during the microwave treatment, indicating that the OMCs and the metal precursor strongly absorb the microwave radiation with temperatures approaching 800–1,000 °C. 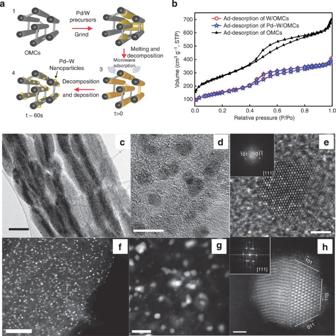Figure 1: Pd–W decorated OMCs. (a) Synthesis diagram of Pd–W decorated OMCs (Pd–W/OMCs) catalysts: (1) OMCs; (2) mixture of Pd and W precursors with OMCs; (3) mixture of partly decomposed metallic precursors and (4) Pd–W/OMCs. (b) Adsorption–desorption isotherms at standard pressure (STP) of OMCs (black triangle), W/OMCs (red circles, which are difficult to observe owing to overlap) and Pd–W/OMCs (blue star). (c) Low-magnification transmission electron microscopy (TEM) image of Pd–W/OMCs. Scale bar, 500 nm. (d) High-magnification TEM image of the Pd–W nanoparticles adsorbed on the carbon support. Scale bar,is 10 nm. (e) Atomic resolution TEM image of one Pd–W nanoparticle acquired by negative Cs imaging technique, where bright spots represent atom columns; several extra bright dots in the image are most probably assigned to Pd dopant atoms. Scale bar, 2 nm. (f–h) High-angle annular dark-field image of Pd–W/OMCs with different magnifications, where the bright spots represent the Pd–W nanoparticles/atoms and the grey regions are the OMCs. Scale bars, 100, 20 and 1 nm inf–h,respectively. Figure 1: Pd–W decorated OMCs. ( a ) Synthesis diagram of Pd–W decorated OMCs (Pd–W/OMCs) catalysts: (1) OMCs; (2) mixture of Pd and W precursors with OMCs; (3) mixture of partly decomposed metallic precursors and (4) Pd–W/OMCs. ( b ) Adsorption–desorption isotherms at standard pressure (STP) of OMCs (black triangle), W/OMCs (red circles, which are difficult to observe owing to overlap) and Pd–W/OMCs (blue star). ( c ) Low-magnification transmission electron microscopy (TEM) image of Pd–W/OMCs. Scale bar, 500 nm. ( d ) High-magnification TEM image of the Pd–W nanoparticles adsorbed on the carbon support. Scale bar,is 10 nm. ( e ) Atomic resolution TEM image of one Pd–W nanoparticle acquired by negative Cs imaging technique, where bright spots represent atom columns; several extra bright dots in the image are most probably assigned to Pd dopant atoms. Scale bar, 2 nm. ( f – h ) High-angle annular dark-field image of Pd–W/OMCs with different magnifications, where the bright spots represent the Pd–W nanoparticles/atoms and the grey regions are the OMCs. Scale bars, 100, 20 and 1 nm in f – h, respectively. Full size image As shown in Fig. 1b , the desorption curves of Pd–W/OMCs and W/OMCs overlap with BET surface areas equal to 536 and 534 m 2 g −1 , respectively, which is significantly lower than that of pure OMCs (~978 m 2 g −1 ). The calculated average pore size is 4.26 nm for Pd–W/OMCs and 4.27 nm for W/OMCs, slightly smaller than for pure OMCs (4.67 nm). Both observations indicate that the OMCs pores are filled with W and Pd metals. Figure 1c shows a low-magnification transmission electron microscopy (TEM) image of Pd–W/OMCs. At higher magnification ( Fig. 1d ), the crystalline Pd–W particles appear dark on the mesoporous carbon support. The Pd–W nanoparticles are found to be crystalline and homogeneously distributed in the OMCs ( Fig. 1d ) with an average diameter of 6.9±1.4 nm. Figure 1e shows an atomic resolution TEM image of one Pd–W particle using the negative Cs imaging technique [31] . The bright spots in the image are atom columns, while the amorphous area around is attributed to the OMCs support. Brighter spots in Fig. 1e could be assigned to Pd dopant atoms in the W-matrix owing to their different electric potential. The image and the fast Fourier transform ( Fig. 1e , inset) clearly indicate that this particle has a body-centered cubic (bcc) structure with a calculated spacing along [110] of 0.23 nm, which agrees well with the W microstructure (PDF no. 040806). In order to elucidate whether the Pd–W nanoparticles are homogeneously alloyed or exhibit a core-shell structure, scanning TEM (STEM) with energy dispersive X-ray spectroscopy (EDS) elemental analysis was used (JEOL ARM200F microscope equipped with probe Cs corrector). The microscope was set to achieve Z-contrast imaging [32] . Large area STEM images are shown in Fig. 1f,g . The bright area represents the Pd–W particles and the grey area corresponds to the OMCs support. Figure 1h shows the atomic resolution Z-contrast image of one Pd–W nanoparticle with bcc structure in the [111] orientation. Different facets of the bcc structure can be clearly observed. Various particles were analysed by nanobeam electron diffraction ( Supplementary Fig. 1 ), which confirm that most particles display a bcc structure. However, we also found a few particles with face-centered cubic structure, probably formed and stabilized in the fast synthesis process (see STEM image in Supplementary Fig. 2 ). The fast synthesis process probably also explains why most Pd–W particles are polycrystalline, as seen in Fig. 1h , where only a fraction of the atoms could be well resolved. Some defects, such as crystal twin boundaries, are also observed in the particles ( Supplementary Fig. 3 ). It should also be noted that even though the particle can be indexed as having the bcc W structure, we observed some lattice distortion in both high-resolution TEM (HRTEM) and STEM images (as fast Fourier transform shows), which could possibly be explained by the presence of Pd atoms causing strain by the atomic lattice mismatch. EDS linescan ( Fig. 2a,b ) and elemental mapping ( Fig. 2c–f ) clearly show that Pd and W are quite homogeneously distributed in the nanoparticles with a Pd:W ratio of 1:8. Also, the atomic resolution STEM images ( Fig. 1h and Supplementary Fig. 4 ) give additional direct proof that the nanoparticles do not display core-shell structures, as evidenced by the absence of direct contrast in the images, as expected for core-shell structures [27] . 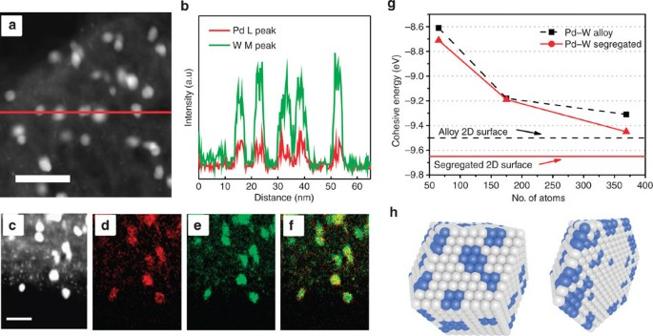Figure 2: Electron microscopy characterization. (a) High-angle annular dark-field image of the Pd–W/OMCs. (b) Intensity profiles of Pd (L) and W (M) components in the Pd–W/OMCs obtained by a energy dispersive X-ray spectroscopy (EDS) line scan analysis (along the red line inafrom left to right). (c) Scanning transmission electron microscopy (STEM) image showing the Pd–W nanoparticles as bright area. (d–f) EDS mapping of the Pd–W/OMCs shown inc, with the signals attributed to the different elements shown as Pd (d), W (e) and their combination (f). (g) Cohesive energy of Pd–W (14% Pd) dodecahedral alloys according to the nanoparticle sizes. (h) A schematic representation of a Pd–W nanoparticle with Pd segregated preferentially at the particle surface, where Pd islands act as catalytic spots for ORR. Grey atoms corresponds to W, and blue atoms to Pd. Scale bars, 20 nm (a,c). Figure 2: Electron microscopy characterization. ( a ) High-angle annular dark-field image of the Pd–W/OMCs. ( b ) Intensity profiles of Pd (L) and W (M) components in the Pd–W/OMCs obtained by a energy dispersive X-ray spectroscopy (EDS) line scan analysis (along the red line in a from left to right). ( c ) Scanning transmission electron microscopy (STEM) image showing the Pd–W nanoparticles as bright area. ( d – f ) EDS mapping of the Pd–W/OMCs shown in c , with the signals attributed to the different elements shown as Pd ( d ), W ( e ) and their combination ( f ). ( g ) Cohesive energy of Pd–W (14% Pd) dodecahedral alloys according to the nanoparticle sizes. ( h ) A schematic representation of a Pd–W nanoparticle with Pd segregated preferentially at the particle surface, where Pd islands act as catalytic spots for ORR. Grey atoms corresponds to W, and blue atoms to Pd. Scale bars, 20 nm ( a , c ). Full size image We use first-principles calculation to investigate the stability and the crystal structure of the synthesized Pd–W nanoparticles. To identify the most stable configuration, we calculate the cohesive energy ( E Coh ) of various W dodecahedral nanoparticles with two different Pd arrangements (an alloy and a segregated state), both systems exhibit a bcc motif and 14% of Pd. The first configuration is obtained by randomly replacing W atoms by Pd, whereas in the second the Pd atoms are segregated into small islands maintaining the bcc structure. The results are depicted in Fig. 2g . As observed, the segregated states are energetically preferred over the alloy configurations, and similar results are obtained for larger systems such as Pd–W surfaces ( Supplementary Fig. 5 ). In addition, we have complemented these studies by calculating the degree of segregation in bimetallic systems according to the procedure used by Greeley and Norskov [33] . The segregation energy ( E Seg ), defined in Methods section, is a useful term that indicates how feasible the segregation of elements in bimetallic systems is. In our case, the resulting E Seg of Pd on the bcc W(110) surface is equal to −1.62 eV, which indicates a strong tendency to surface segregation. Negative E Seg is common for Cu, Pd, Ag, Pt and Au solutes that generally segregate strongly to the surface in a variety of hosts. These calculations, supported by the HRTEM images in Fig. 1 strongly suggests that the Pd–W nanoparticles are constituted of small Pd islands, preferentially located at the surface, in a matrix of a W bcc structure, a schematic representation is depicted in Fig. 2h . The segregation of Pd into small islands is also further supported by the phase diagram of Pd–W, which shows that Pd is only able to form homogeneous alloys for Pd/W ratios up to only ~0.02 (at 1,200 K; ref. 34 ), which is far below our determined ratios of Pd/W ratio of 0.13. X-ray photoelectron spectroscopy (XPS) of bare OMCs and metal-loaded OMCs ( Fig. 3a ) confirm the presence of both Pd and W for Pd–W/OMCs, only W for W/OMCs, and no metals for the non-decorated OMCs. In this case, the Pd:W atomic ratio determined for the Pd–W/OMCs sample is 1:7.9, which matches perfectly with the data from microarea EDS analysis, supporting a homogenous sample composition. The C 1 s spectrum of Pd–W/OMCs is typical for carbon in sp 2 hybridization with a pronounced ‘tailed’ structure and a π – π * excitation feature at 290.3 eV (ref. 35 ). The O 1 s spectrum in Fig. 3c shows three types of oxygen at 530.6, 532.0 and 533.6 eV, corresponding to W–O, W–OH (and, probably, double C=O bond) and organic C–OH bond, respectively. The W 4 f spectrum can be fitted by three doublets with the binding energies (BEs) of the W 4 f 7/2 component at 31.8, 32.7 and 35.5 eV, respectively. These are attributed to metallic W, W carbide and WO 3 (ref. 36 ), which are in good agreement with powder X-ray diffraction data ( Supplementary Fig. 6 ). Several important conclusions can be drawn from the analysis of the XPS spectra. The W carbide signal probably originates from the interface between the Pd–W nanoparticle and the OMCs support, suggesting a good contact interface that may improve the electrochemical performance owing to a good electron conduction from the active nanoparticles to the carbon support, as well as lead to an improved stability of the nanoparticles by hindering their agglomeration. The good anchoring and long-term stability are supported by measuring the size distribution of the Pd–W nanoparticles before and after the electrochemical testing ( Supplementary Fig. 7 ). The BE attributed to metallic W in both W/OMC and Pd–W/OMC samples (31.8 eV) is slightly higher than corresponding value for the bulk metal (31.4 eV), which seems to be related to nanoparticle size effect ( Fig. 3f ). Addition of Pd results in an increase of WO 3 contribution ( Fig. 3e,f ) that indicates direct reduction of Pd (II) ions by metallic W, thus confirming the incorporation of Pd atoms into the W nanoparticle. Correspondingly, Pd 3 d spectrum of Pd–W/OMCs ( Fig. 3d ) demonstrates only one chemical state of Pd atoms with BE of Pd 3 d 5/2 at 335.8 eV. This is 0.7 eV higher than the corresponding BE of bulk Pd (0) (335.1 eV), which most likely is owing to a combination of a ‘nanoparticle size effect’ as well as the embedment of the Pd atoms in the W-matrix. The metallic character of Pd is strongly supported by Fig. 3g , which shows the Pd L 2,3 edge measured by electron energy loss spectroscopy (EELS) for Pd–W/OMC and two reference spectra of Pd and PdO standard materials (DigitalMicrogaph software, E. A.). From the spectra, it is clear that metallic Pd does not have strong L 2,3 peaks, opposite to PdO. The Pd L 2,3 spectrum of Pd–W/OMCs exhibits features similar to metallic Pd, strongly suggesting a metallic nature of the Pd islands in the Pd–W particles. Unambiguous confirmation of the metallic nature of the Pd atoms is also obtained by performing EXAFS studies at the Shanghai Synchrotron Radiation Facility. Supplementary Fig. 8 shows the Pd–K edge of the two different Pd–W/OMC samples (one fresh and one sample stored at ambient conditions for 18 months) together with a reference Pd foil sample. It is evident from Supplementary Fig. 8 that the Pd–K edge of both Pd–W/OMC samples exhibit metallic character very similar to that of the Pd foil. After data analysis using the Artemis programme in the IFEFFIT software package, we fit the Fourier transformation of the k -weighted EXAFS oscillations by a Pd–Pd model. 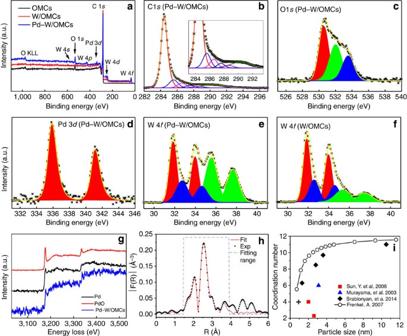Figure 3: Elemental analysis of Pd–W/OMCs. (a) X-ray photoelectron spectroscopy (XPS) spectra of the W/OMCs (red line), Pd–W/OMCs (blue line) and pristine OMCs support (black line). High-resolution XPS spectra of the as prepared Pd–W/OMCs hybrid C 1s(b), O 1s(c), Pd 3d(d) and W 4f(e) photoelectron lines. (f) W 4fspectrum of the W/OMCS composite synthesized using the same method as Pd–W/OMCs. (g) Electron energy loss spectroscopy (EELS) analysis. (h) Fourier transforms |F(R)| ofk·χ(k) obtained by the Δk interval 2.1–12.2 Å−1. The red line shows the fitted function to the experimental values (black dots). (i) Coordination number (N) versus Pd particle sizes, solid squares50, triangles51and diamonds37represent experimental values of ‘N’ for various Pd nanoparticles obtained from given references. The open circles indicate the theoretical coordination number of cuboctahedral PdXclusters calculated at different shell sizes(from 1 (Pd13) to 25 shells (Pd55301)) in accordance to Frenkelet al.38In our case, the Pd–W/OMC sample exhibit aN=4, indicating a Pd agglomeration in the range of 1–2 nm (indicated with a cross), which may suggest the presence of islands up to 20 atoms, see alsoSupplementary Fig. 9. Figure 3h shows the k·χ ( k ), from k space to R space over the range of 2.1–12.2 Å −1 to obtain a radial distribution function and the corresponding fit to the experimental data. It is clear that a Pd–Pd model gives a very good agreement with the experimental data. Even more importantly, the EXAFS data can be used to derive the coordination number of Pd atoms, which represents the average number of Pd neighbours for each Pd atom. Supplementary Table 1 shows that our Pd–W/OMC sample exhibit a coordination number of 4.0 (±0.3). This is a quite remarkable value. Figure 3i shows a collection of coordination numbers of related Pd systems. In particular, a systematic study by Srabionyan et al. [37] for Pd clusters on Al 2 O 3 and theoretical calculations for small Pd clusters by Frenkel et al. [38] indicates that a coordination number of 4 is consistent with Pd islands being ~1 nm across. Modelling the coordination number for different configurations ( Supplementary Fig. 9 ) shows that our Pd islands contain ~10–20 atoms, and that they indeed are segregated into islands at the surface of the Pd–W particles. It is also clear that such low coordination number in a nanoparticle cannot be achieved considering neither a core-shell structure nor a homogeneous Pd–W alloy, but rather strongly indicates a Pd island configuration. The fact that the Pd atoms have metallic nature further shows that they are situated in a reducing W environment. Earlier studies show that without a reducing environment, such small clusters would undoubtedly be oxidized [39] . Figure 3: Elemental analysis of Pd–W/OMCs. ( a ) X-ray photoelectron spectroscopy (XPS) spectra of the W/OMCs (red line), Pd–W/OMCs (blue line) and pristine OMCs support (black line). High-resolution XPS spectra of the as prepared Pd–W/OMCs hybrid C 1 s ( b ), O 1 s ( c ), Pd 3 d ( d ) and W 4 f ( e ) photoelectron lines. ( f ) W 4 f spectrum of the W/OMCS composite synthesized using the same method as Pd–W/OMCs. ( g ) Electron energy loss spectroscopy (EELS) analysis. ( h ) Fourier transforms |F(R)| of k·χ ( k ) obtained by the Δk interval 2.1–12.2 Å −1 . The red line shows the fitted function to the experimental values (black dots). ( i ) Coordination number ( N ) versus Pd particle sizes, solid squares [50] , triangles [51] and diamonds [37] represent experimental values of ‘ N ’ for various Pd nanoparticles obtained from given references. The open circles indicate the theoretical coordination number of cuboctahedral Pd X clusters calculated at different shell sizes(from 1 (Pd 13 ) to 25 shells (Pd 55301 )) in accordance to Frenkel et al. [38] In our case, the Pd–W/OMC sample exhibit a N =4, indicating a Pd agglomeration in the range of 1–2 nm (indicated with a cross), which may suggest the presence of islands up to 20 atoms, see also Supplementary Fig. 9 . Full size image Electrochemical characterization ORR catalytic activity was tested by loading identical mass amounts of our materials onto glassy carbon electrodes. According to cyclic voltammetry (CV) in O 2 saturated 0.1 M KOH, W/OMCs (prepared by the same method as Pd–W/OMCs) exhibited very poor ORR activity ( Fig. 4a , red line). The ORR peak potential of W/OMCs appears at 0.69 V, much lower than that of Pt/Vulcan catalyst (~0.77 V; Fig. 4a , black line). In contrast, the ORR peak potential of Pd–W/OMCs modified electrode is ~0.75 V, very close to the value for commercial 60% Pt/Vulcan catalyst. The ORR onset potential of Pd–W/OMCs (~0.86 V) is positively shifted by 60 mV compared with the W/OMCS composite. Although the onset potential is lower than that of Pt/Vulcan catalyst (~0.97 V), it is clear that the small amount of Pd in the Pd–W nanoparticles has a significant effect on the ORR performance. CV experiments performed in neutral and acidic electrolytes give similar trends and are shown in Supplementary Fig. 10 . To verify the ORR catalytic pathways of the hybrid materials, the formation of peroxide species (HO 2 − ) during the ORR process was monitored by rotating ring-disk electrode (RRDE) measurements ( Fig. 4b ). The limiting ORR current declines slightly in the potential scan at potentials lower than 0.6 V. This is explained by considering that W nanoparticles and other active sites take part in the ORR as two-electron ( e ) catalytic processes leading to the production of more hydrogen peroxide, which will prevent the direct 4 e production of diffused oxygen molecules at the Pd catalyst. The measured HO 2 − yields are above 60% for W/OMCs and lower than 16% for Pd–W/OMCs, respectively, over the potential region of 0.3–0.65 V. The derived electron transfer numbers at 0.6 V are 2.67 for W/OMCs and 3.89 for Pd–W/OMCs, respectively ( Fig. 4c ), indicating an efficient ORR process that is very close to the direct 4 e process obtained with the commercial 60% Pt/Vulcan sample. 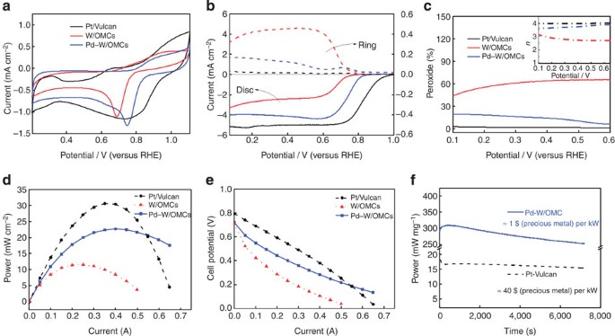Figure 4: Electrochemical characterization Pd–W/OMCs. (a) CV curves of commercial Pt/Vulcan (black line), W/OMCs (red line) and Pd–W/OMCs (blue line), showing that Pd doping positively shifts the reduction potential of oxygen at the W/OMCs modified electrode and increases the current intensity of ORR. Potentials are specified with reversible hydrogen electrode (RHE) as reference. (b) Polarization curves of ring (dotted line) and disc (solid line) electrodes at 1,600 r.p.m. by coating Pt/Vulcan (black), W/OMCs (red) and Pd–W/OMCs (blue) onto disc electrode, scan rate: 10 mV s−1. (c) Percentage of peroxide (solid line) and the electron transfer number (n; inset, dotted line) of Pt/Vulcan (black), W/OMCs (red) and Pd–W/OMCs at various potentials, based on the corresponding RRDE data inb. (d) Fuel cell performance plots for different cathode with the same metal loading at an accessed Pd/Vulcan coated anode (black circles: Pt/Vulcan, blue square: Pd–W/OMCs, red triangle: W/OMCs) using 3 M formic acid as fuel and electrolyte, non-humidified 5 bar oxygen as oxidant. (e) Corresponding I–V curves of the fuel cell ind. (f) Power output per milligram (precious metal) of the fuel cell over time using Pt/Vulcan (dashed line) and Pd–W/OMCs as cathode materials. Figure 4: Electrochemical characterization Pd–W/OMCs. ( a ) CV curves of commercial Pt/Vulcan (black line), W/OMCs (red line) and Pd–W/OMCs (blue line), showing that Pd doping positively shifts the reduction potential of oxygen at the W/OMCs modified electrode and increases the current intensity of ORR. Potentials are specified with reversible hydrogen electrode (RHE) as reference. ( b ) Polarization curves of ring (dotted line) and disc (solid line) electrodes at 1,600 r.p.m. by coating Pt/Vulcan (black), W/OMCs (red) and Pd–W/OMCs (blue) onto disc electrode, scan rate: 10 mV s −1 . ( c ) Percentage of peroxide (solid line) and the electron transfer number ( n ; inset, dotted line) of Pt/Vulcan (black), W/OMCs (red) and Pd–W/OMCs at various potentials, based on the corresponding RRDE data in b . ( d ) Fuel cell performance plots for different cathode with the same metal loading at an accessed Pd/Vulcan coated anode (black circles: Pt/Vulcan, blue square: Pd–W/OMCs, red triangle: W/OMCs) using 3 M formic acid as fuel and electrolyte, non-humidified 5 bar oxygen as oxidant. ( e ) Corresponding I–V curves of the fuel cell in d . ( f ) Power output per milligram (precious metal) of the fuel cell over time using Pt/Vulcan (dashed line) and Pd–W/OMCs as cathode materials. Full size image We test our catalyst in real-life applications by implementing the Pd–W/OMCs as cathode ORR catalysts in a direct formic acid fuel cell system. The results are depicted in Fig. 4d where the power output of the Pd–W/OMCs modified electrode is slightly lower but yet comparable to Pt/Vulcan. We also note that it is possible to draw larger currents in the Pd–W/OMCs case, suggesting a lower resistance of the membrane electrode assembly, probably originating to the formation of WC at the interface of the OMCs and the Pd–W catalyst as discussed earlier. Above 0.4 A, the reaction becomes diffusion-limited in the case of Pt/Vulcan, visible by a deviation from the linear range, resulting in a decreasing cell potential. This effect is not visible for W/OMCs or Pd–W/OMCs. The ORR for W/OMCs and Pd–W/OMCs is strongly dependent on the potential, indicated by an almost complete absence of a linear range, as observed in several reports [40] , [41] . The very good activity of Pd–W/OMCs is rather astonishing considering the fact that the Pt/Vulcan reference system was chosen such that the total weight of Pt corresponded to the total weight of Pd plus W in our material. The deactivation stability test shows that Pd–W/OMCs is comparable to Pt/Vulcan. Pd–W/OMCs deactivates by 18% and Pt/Vulcan by 9% after 2 h when drawing a maximum current. We noted, however, that under less extreme conditions, tested by CV, our Pd–W/OMCs shows negligible decrease in catalytic activity after ~54 h of continuous testing ( Supplementary Fig. 11 ). This is further manifested by statistical analysis of TEM images of Pd–W/OMCs samples after CV tests, which shows an identical size distribution as before the electrochemical tests with no sign of agglomeration or catalyst leakage, which is different from the commercial catalysts that showed clear signs of agglomeration ( Supplementary Fig. 7 ). The high electrochemical stability indicates a preservation of the nanoparticle morphology in line with the molecular dynamics (MD) studies of our Pd–W nanoparticles, which shows no migration of the Pd atoms in the W-matrix at room temperature ( Supplementary Fig. 12 ), similarly the EXAFS and EELS data also confirm a metallic character of the Pd islands after more than 18 month of storage at ambient conditions. The most advantageous attributes of our catalyst materials are however revealed by comparing the activity per milligrams of noble metal in fuel cell tests, which shows that the Pd–W/OMCs catalyst clearly outruns the Pt/Vulcan-based catalyst. Figure 4f shows the power output per milligrams (noble metal) over time. Considering only the metal (Pt, Pd and W) prize per kilowatt (US$ per kW) of the newly designed Pd–W/OMCs catalysts, we derive a cost of ~1 US$ per kW, compared with ~40 US$ per kW for the commercial Pt-based catalyst. We also point out that our synthesis method is versatile, and that a similar ORR performance is obtained for both Pd–W nanoparticles supported on helical carbon nanofibres and Vulcan ( Supplementary Fig. 13 ). Evidently, the cost of the latter support is significantly lower than OMCs, which is prepared by template methods. It is clear that the Pd–W nanoparticles exhibit an extraordinarily good ORR activity considering the low amount of Pd in the structure. Theoretical calculations To understand our previous results, we have studied the ORR process on Pd–W nanoparticles by means of DFT. Using the dissociative mechanism and the computational hydrogen electrode (CHE) [42] , we analysed the ORR performance on dodecahedral Pd–W clusters (Pd 24 W 151, bcc structure) with a Pd:W ratio of 1:7, which is close to our experimental composition. We built seven different Pd 24 W 151 clusters, and we identified ten catalytic sites composed of W 3 , Pd–W 2 , Pd 2 W, Pd 3 and Pd 4 atomic islands, located at the centre and at the edge of a crystal facet, the clusters are depicted in Fig. 5a and Supplementary Fig. 14 . We first calculated the adsorption energy of O* and HO* intermediates on the diverse catalytic sites. Afterwards, we computed the change in Gibbs free energy (Δ G ) during ORR at equilibrium potential of U 0 =1.23 V, which allows to identify the rate-limiting step, the ORR overpotential and subsequently the catalyst activity. Here, ORR ( Fig. 5b ) is initiated by the adsorption of ½ O 2 on the catalytic site (Pd 4 island), and then followed by the transfer of two proton–electron (H + +e − ) pairs generating and releasing one water molecule. Similarly, we studied the ORR performance on all other catalytic sites shown in Fig. 5a and Supplementary Fig. 14 . The change in Δ G during ORR performed on a Pd 4 island is depicted in Fig. 5c , similar results are obtained for other configurations (detailed description is given in Supplementary Note 1 , Supplementary Fig. 14 and Supplementary Fig. 15 ). The activity Volcano plot is shown in Fig. 5d , where the ORR activity for different catalytic sites on the Pd 24 W 151 nanoparticle is plotted against O adsorption energy (Δ E O ). Interestingly, we observe that a slight segregation of Pd atoms into three or larger atomic islands can significantly boost the ORR activity of these sites, leading some Pd sites (Pd 3 and Pd 4 island at the facet centre) to exhibit a catalytic activity higher than Pd(111) and similar to Pt(111) periodic surfaces. The improved mechanism is similar to the synergistic effects observed in other core-shell particles, where the weaker interaction of oxygenated species at the Pd islands results in lower ORR overpotential and thus improved catalytic activity, which is consistent with our experimental observations. 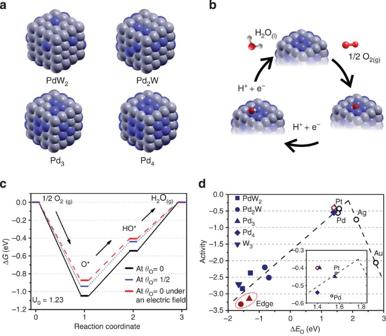Figure 5: DFT studies of the ORR on Pd islands. (a) Geometrically optimized structures showing the Pd–W nanoparticles with Pd–W2, Pd2W, Pd3and Pd4catalytic sites (Pd blue, W grey). (b) Oxygen reduction scheme used to study the catalytic activity (O red and H white). (c) Change in Gibbs free energy during ORRs performed on a Pd4island of the Pd–W cluster at two different oxygen coverage, zero (θO=0) and half of a monolayer (θO=1/2), and under the effect of the electric field generated by the solvent, see alsoSupplementary Figs 15–17. The ORR is initiated by the adsorption of ½ O2on the catalytic site, followed by the transfer of two proton–electron (H++e−) pairs, that results in the formation and release of one water molecule. (d) Activity volcano plot for diverse catalytic sites in Pd24W151nanoparticles. The activity of catalytic sites located at the center of the particle facet is in blue, whereas red indicates islands at the edge. Pt, Pd, Ag and Au periodic surfaces (open circles) are shown for comparison, information taken from ref.42. The inset shows the ORR activity of the materials near the top of the volcano, the red-open-diamond indicates the activity of a Pd4island considering the effect of the solvent. The dashed line is a guide to the eyes. Figure 5: DFT studies of the ORR on Pd islands. ( a ) Geometrically optimized structures showing the Pd–W nanoparticles with Pd–W 2 , Pd 2 W, Pd 3 and Pd 4 catalytic sites (Pd blue, W grey). ( b ) Oxygen reduction scheme used to study the catalytic activity (O red and H white). ( c ) Change in Gibbs free energy during ORRs performed on a Pd 4 island of the Pd–W cluster at two different oxygen coverage, zero ( θ O =0) and half of a monolayer ( θ O =1/2), and under the effect of the electric field generated by the solvent, see also Supplementary Figs 15–17 . The ORR is initiated by the adsorption of ½ O 2 on the catalytic site, followed by the transfer of two proton–electron (H + +e − ) pairs, that results in the formation and release of one water molecule. ( d ) Activity volcano plot for diverse catalytic sites in Pd 24 W 151 nanoparticles. The activity of catalytic sites located at the center of the particle facet is in blue, whereas red indicates islands at the edge. Pt, Pd, Ag and Au periodic surfaces (open circles) are shown for comparison, information taken from ref. 42 . The inset shows the ORR activity of the materials near the top of the volcano, the red-open-diamond indicates the activity of a Pd 4 island considering the effect of the solvent. The dashed line is a guide to the eyes. Full size image We finally consider how solvation potential and the effect of oxygen coverage on the W surface (which might be very likely as indicated by the experimental data) might have on the catalytic activity of the Pd islands. To investigate this, we performed the same calculations as above but at two different oxygen coverage, zero ( θ O =0) and half of a monolayer ( θ O =1/2), on the W surface ( Supplementary Fig. 16 ) and also investigated the effect of the electric field generated by a solvent ( Supplementary Fig. 17 ). In both cases, the change in the η ORR is <0.15 V, and considering that the η ORR variation will be similar in all other studied configurations, the trend in catalytic activity ( Fig. 5d ) is not significantly modified, which is in line with earlier reports [43] . We note however that a deep understanding of how solvation effects might influence the kinetics of the oxygen reduction process would require a more thorough analysis. Such extensive analysis is out of scope for this paper, but work is in progress to address this in a later study. To conclude, we have shown that by a simple microwave-assisted synthesis, we are able to produce highly dispersed small Pd–W nanoparticles supported on OMCs. Although the concentration of Pd in the Pd–W nanoparticles is as low as 14 at.%, we show that this new hybrid material exhibits excellent properties for ORR in electrochemical and fuel cell tests. We explain the good catalytic properties by a slight segregation of Pd in the Pd–W nanoparticles leading to the formation of Pd islands, 10–20 atoms large, which is unambiguously confirmed by a coordination number analysis of EXAFS data. The enhanced ORR activity originates from two advantageous properties of the Pd–W/OMC composite; (i) a synergistic effect from the W environment on the Pd atoms, leading to catalytic hotspots for certain atomic configurations, as supported by DFT calculations, and (ii) a reducing environment for the Pd islands imposed by the W environment leading to metallic character of the Pd atoms, even after 18 months of storage at ambient conditions, as confirmed by EXAFS and EELS studies. Our hybrid material can be implemented as fuel cell cathode electrocatalysts giving a power output at a price of 1 US$ per kW (based on the amount of precious metal). This is roughly 40 times lower than the corresponding value of a commercial 60% Pt/Vulcan cathode. Finally, our results show a new way for nanoparticle design, which in many cases, are simpler than the corresponding core-shell structures. The presented mechanism of how the formation of few-atomic noble metal islands can strongly enhance the ORR activity makes the study interesting not only for fundamental scientific reasons but evidently also has a high technological impact. Pd–W/OMCs synthesis OMCs were synthesized according to a classic hard-template method. An amount of 6.0 mg Pd acetate (Sigma-Aldrich, 99% in purity), 60 mg W hexacarbonyl (Sigma-Aldrich, 97% in purity) and 50 mg OMCs were mixed together and ground for 3 min. A volume of 1 ml toluene was then added into the mortar followed by an additional 3 min grinding. The mixed suspension was kept in a fume hood at room temperature until it was completely dry. The mixture was then transferred into a round-bottom quartz boat, put into a kitchen microwave oven (Novaline, Power output: 700 W, 2.45 GHz) and purged with argon at a flow rate of 100 ml min −1 for 3 h. Thereafter, a full-power microwave treatment was performed for 1 min. The microwave-treated composite was cooled down to room temperature and collected as Pd–W/OMCs. The W/OMCs composite was synthesized according to a similar method without adding the Pd precursor. Characterization HRTEM analysis was performed with a FEI Titan G2 60–300 microscope equipped with an image spherical aberration (Cs) corrector operated at 300 kV. The atomic resolution STEM images and EDS elemental analysis were obtained from JEOL ARM200F microscope equipped with probe Cs corrector. XPS spectra were recorded with Axis Ultra DLD electron spectrometer (Kratos Analytical Ltd, UK). A monochromated Al K α source operated at 150 W and a hybrid lens system with a magnetic lens, providing an analysis area of 0.3 × 0.7 mm, were used for the measurements. Before the measurements, BE scale was calibrated in accordance with ISO/TC 201 Standard: ISO 15472:2010—‘X-ray photoelectron spectrometers—Calibration of energy scales’, using corresponding photoelectron lines of Au 4 f 7/2 (at 83.96 eV), Ag 3 d 5/2 (at 368.21 eV) and Cu 2 p 3/2 (at 932.62 eV). Owing to a good conductivity of the samples, a charge neutralization system was not used, and experimentally measured BEs did not require an additional calibration. High-resolution XPS spectra (C 1 s , O 1 s , Pd 3 d and W 4 f ) were substracted with a Shirley background and fitted using a linear combination of 70:30 Gauss–Lorentz functions, while asymmetrical functions were applied to fit Pd 3 d line and main component of C 1 s spectrum. Pd 3 d and W 4 f doublets were constrained with corresponding spin-orbit splitting and intensity ratio of the doublet’s components. Processing of the spectra was accomplished with the Kratos software. Direct formic acid fuel cell system test were conducted in a 5- cm 2 quickCONNECT cell fixture from Quintech with carbon serpentine flow fields at 30 °C cell and fuel temperature. Surface area of the Pd–W/OMCs and W/OMCs were determined by Micromeritics TriStar II 3020 instrument (Micromeritics Instrument Corp.), using N 2 adsorption at 77 K. Before electrochemical testing, the glassy carbon electrode (diameter 5 mm) was polished with 0.05 mm aluminium oxide powder and then cleaned by ultrasonication in acetone, ethanol and water, respectively. Six microlitres catalyst inks (5 mg ml −1 ) were drop cast onto the pretreated glassy carbon surface and dried in air. CV and RRDE tests were recorded on a Autolab PGSAT-302N potentiostat/galvanostat connected to a rotating electrode system (Pine, USA) with Ag/AgCl as reference electrode and a platinum rod as counter electrode. The working electrode was scanned in 0.1 M KOH solution by successive (CV) and line sweep voltammetry (LSV) at 0.05 V s −1 in the potential region 0.2–1.1 V. Before CV and RRDE tests, the alkaline solution was bubbled with oxygen for >30 min. The current densities in both CV and RRDE data were normalized according to the geometric area of the glassy carbon disc. EXAFS measurements at Pd–K edge in both transmission (for a pure Pd foil) and fluorescence (for the Pd–W sample) mode were performed at the BL14W1 in Shanghai Synchrotron Radiation Facility. The electron beam energy was 3.5 GeV and the stored current was 240 mA (top-up). A 38-pole wiggler with the maximum magnetic field of 1.2 T inserted in the straight section of the storage ring was used. XAFS data were collected using a fixed-exit double-crystal Si(311) monochromator. A 32-element Ge solid-state detector was used to collect the fluorescence signal, and the energy was calibrated using Pd foil and a third ionization chamber. The photon flux at the sample position was 7.2 × 10 11 photons per second. The raw data analysis was performed using IFEFFIT software package according to the standard data analysis procedures [44] .The spectra were calibrated, averaged, pre-edge background subtracted and post-edge normalized using Athena programme in IFEFFIT software package. The Fourier transformation of the k -weighted EXAFS oscillations, k·χ ( k ), from k space to R space was performed over a range of 2.1–12.2 Å −1 to obtain a radial distribution function, then the data fitting was performed by Artemis programme in IFEFFIT. Theoretical calculations DFT calculations were performed using the SIESTA code [45] within the local density approximation [46] . Electron exchange-correlation functionals are represented with the generalized gradient approximation and the Perdew, Burke and Ernzerhof model [47] for the non-local corrections. The wave functions for the valence electrons are represented by a linear combination of pseudo-atomic numerical orbitals [48] using double-ζ plus one polarized orbital. The real-space grid used for charge and potential integration is equivalent to a plane wave cutoff energy of 350 Ry. All systems are fully geometrically relaxed before and during both adsorption events, and no constrains were applied at any moment until the maximum forces were <0.04 eV per Å. Ab initio MD simulation were carried out on four different W dodecahedral clusters (Pd 24 W 151 , 14% Pd) with Pd islands. We performed the MD at temperature equal to 300±10 K during 1.6 ps using a time step of 1 fs for the integration of the equations of motion. The temperature was controlled by Nose thermostat with a Nose [49] mass equal to 50 Ry × fs 2 by using the Siesta code. Free energies of intermediates in electrochemical reactions were calculated based on the CHE model [42] . The CHE model defines that at standard conditions (pH=0 in the electrolyte and 1 bar of H 2 in the gas phase at 298.15 K), the chemical potential of a proton–electron pair (H + +e − ) in solution is equal to half of the chemical potential of a gas-phase H 2 molecule. The Gibbs free energy change (Δ G 0 ) of intermediates is calculated by Δ G 0 =Δ E +ΔZPE— T Δ S , where Δ E is the energy change obtained from DFT calculations (O or OH adsorption energy, relative to gas-phase H 2 O and H 2 molecules), ΔZPE is the change in zero point energies, T is temperature (298.15 K), and Δ S is the change in entropy, these values were taken fromref. [42] . The effect of a bias on states involving electrons transfer results in a direct shift in the free energy of the electrons, and it can be included by correcting the Gibbs free energy (Δ G U ) by – e U, where U is the applied bias and e is the number of electrons transferred. The free energy as a function of the applied bias is given by Δ G =Δ G 0 +Δ G U . The cohesive energy is defined as E Coh =( E Total − N W E W − N Pd E Pd )/ N Total , where N W ( N Pd ) indicates the number of W (Pd) atoms, E W ( E Pd ) indicates the energy of an isolated W (Pd) atom. E Total is the final energy of the optimized Pd–W nanoparticle containing N Total atoms. The segregation energy is defined as E Seg = E A/B −( E B/B − E B,bulk ), where E A/B is the energy of Pd atom at the top layer in a W(110) surface. E B/B is the energy of a clean W(110) surface, and E A/B,bulk is the energy of a Pd atom embedded in bulk W. How to cite this article: Hu, G. et al. Small palladium islands embedded in palladium–tungsten bimetallic nanoparticles form catalytic hotspots for oxygen reduction. Nat. Commun. 5:5253 doi: 10.1038/ncomms6253 (2014).